Gene-associated markers provide tools for tackling illegal fishing and false eco-certification Illegal, Unreported and Unregulated fishing has had a major role in the overexploitation of global fish populations. In response, international regulations have been imposed and many fisheries have been 'eco-certified' by consumer organizations, but methods for independent control of catch certificates and eco-labels are urgently needed. Here we show that, by using gene-associated single nucleotide polymorphisms, individual marine fish can be assigned back to population of origin with unprecedented high levels of precision. By applying high differentiation single nucleotide polymorphism assays, in four commercial marine fish, on a pan-European scale, we find 93–100% of individuals could be correctly assigned to origin in policy-driven case studies. We show how case-targeted single nucleotide polymorphism assays can be created and forensically validated, using a centrally maintained and publicly available database. Our results demonstrate how application of gene-associated markers will likely revolutionize origin assignment and become highly valuable tools for fighting illegal fishing and mislabelling worldwide. Commercially important fish populations worldwide have been overexploited and require rebuilding [1] , [2] . Tight regulations are needed to meet future marine fisheries and conservation objectives. Spatially explicit quotas and closures are common management actions for restoring fish populations and promoting sustainable 'ecosystem-based fisheries management' [3] . Illegal, unreported and unregulated (IUU) fishing poses a major threat to sustainable fisheries, constituting approximately one-fifth of the global catch [4] , [5] . Accordingly, international rules and laws, such as the recent European Commission Control [6] and IUU Regulation [7] , which require catch certificates that state the origin of all fish and fish products traded within the European Union, have been instated.Likewise, consumer awareness regarding vulnerability of fish stocks has been growing, and many local fisheries have been awarded, or are seeking sustainability certification ('eco-labelling') by organizations such as the Marine Stewardship Council (MSC) [8] , despite recent concerns of mislabelling [9] . To enforce fisheries regulations and conservation measures spatially and to provide independent control of catch certificates and mislabelling, forensically validated high-throughput identification methods, tracing individual fish to area/population of origin, are urgently needed. Many tests have been developed to identify the population of origin of fish and fish products [10] , which may be applied singly or in combination to address the generally low statistical power of any individual method. However, many such tests have been hampered by limited tissue availability or quality, especially in processed seafood. In addition, inter-laboratory standardization of operating procedures is inherently difficult and compromises forensic validation [11] . DNA-based tools offer a universal method for assigning fish and fish products to population of origin. DNA is found in all cells in all organisms and can be analysed in any tissue type, from freshly caught fish to a fried fillet. Till now, DNA-based population assignment of marine fish has almost exclusively relied on so-called 'neutral' genetic markers, compromised by weak population-level genetic signatures [12] . Such patterns coincide with the general lack of obvious physical barriers in the sea and typically large effective population sizes of marine fishes [13] . In contrast to population diversification by neutral genetic drift, evolution by natural selection proceeds more rapidly in large populations [14] . To identify genomic regions under divergent selection among natural populations, comparison of genetic differentiation for hundreds or thousands of genetic markers, so-called 'genome scans' are increasingly being used [15] . Genome scans identify genetic markers with highly elevated divergence among populations that do not conform to statistical expectations based on a neutral genetic model. Accordingly, these markers are likely to be located within genomic regions with one or more gene loci under selection. Application of markers randomly distributed across the genome has generally provided a relatively low percentage of these high differentiation outliers putatively subject to selection [16] . Thus, targeting gene-associated markers, has been advocated as it increases the probability of identifying footprints of selection [16] , [17] , [18] . Many marine fish experience divergent environmental conditions, giving ample opportunity for heritable local adaptation [19] , [20] . Locally adapted genes will commonly display more divergent allele frequencies among populations than neutral markers and therefore display markedly elevated power for population assignment [12] . A relatively low number of genes with high genetic differentiation have been identified in marine fish to date, and even fewer used for population assignment [12] . Consequently, targeted identification of suites of gene-associated markers likely affected by direct or indirect 'hitch-hiking', selection will vastly enhance our ability to determine the population of origin of individual marine fish and elucidate their temporal and spatial dynamics. We applied this new population genomics approach to four commercially important marine fish species: Atlantic cod ( Gadus morhua ), Atlantic herring ( Clupea harengus ), sole ( Solea solea ) and European hake ( Merluccius merluccius ), each threatened by overfishing and IUU activities. From extensive sample data-bases ( Fig. 1a-d ), policy-led scenarios of illegal fishing and/or mislabelling were selected for all four species. We demonstrated application of single nucleotide polymorphism (SNP) tools across different geographical scales and in comparison to previously published methods. (1) Cod: Northeast Arctic and Eastern Baltic cod populations thrive, whereas North Sea cod need rebuilding [21] . Strict spatially based landing regulations are in place. Northeast Arctic and Eastern Baltic cod fisheries are MSC-certified. With the proximity and highly divergent status of these major cod populations, there is a large potential for fraud and mislabelling. (2) Herring: no current method can distinguish North Sea from Northeast Atlantic herring (mainly 'Norwegian spring' and 'Icelandic summer spawners'). Tracing the geographical origin of herring is important to MSC for certifying fisheries. (3) Sole: most sole stocks of the Northeast Atlantic Ocean are in the process of rebuilding from high fishing mortalities. It is suspected that a proportion of sole landings in Belgian ports claimed to originate from the Irish Sea/Celtic Sea are, in fact, caught en route between the Irish Sea and the southern North Sea (Thames/Belgian coast), which is closer to market, but closed to fishing. (4) Hake: fishing regulations for hake differ between the Mediterranean and the Atlantic, with legal size limits of 20 cm and 27 cm, respectively. Undersized Atlantic hake are misreported as of Mediterranean origin. 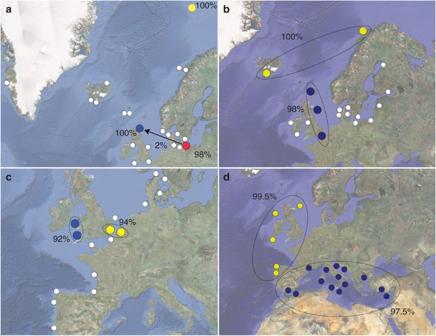Figure 1: Map of sampling localities. Locations for the genetic baselines (white circles) and policy-led individual assignment case studies (coloured circles) for the four commercially important marine species. Shown is the percentage of fish assigned to the sample/area of origin and to other samples/areas (arrows). (a) Atlantic cod (G.morhua) case study: Northeast Arctic cod (yellow), North Sea cod (blue), Baltic cod (red). (b) Atlantic herring (C. harengus) case study: Northeast Atlantic herring (yellow), North Sea herring (blue). (c) Sole (S.solea) case study: Irish Sea/Celtic Sea sole (blue), Thames/Belgian Coast (yellow). (d) European hake (M.merluccius) case study: Mediterranean hake (blue), Atlantic hake (yellow). Figure 1: Map of sampling localities. Locations for the genetic baselines (white circles) and policy-led individual assignment case studies (coloured circles) for the four commercially important marine species. Shown is the percentage of fish assigned to the sample/area of origin and to other samples/areas (arrows). ( a ) Atlantic cod (G. morhua ) case study: Northeast Arctic cod (yellow), North Sea cod (blue), Baltic cod (red). ( b ) Atlantic herring ( C. harengus ) case study: Northeast Atlantic herring (yellow), North Sea herring (blue). ( c ) Sole ( S . solea ) case study: Irish Sea/Celtic Sea sole (blue), Thames/Belgian Coast (yellow). ( d ) European hake (M. merluccius ) case study: Mediterranean hake (blue), Atlantic hake (yellow). Full size image Cod From 21 geographical samples of Eastern Atlantic cod, the genome-scan method identified 132 high differentiation outlier SNPs likely to be influenced by selection out of 1,262 variable and successfully genotyped loci ( Fig. 1a ). For the case scenario of Northeast Arctic, North Sea and Baltic Sea cod, a total of 69 out of 1,120 loci showed signs of being affected by divergent selection ( Fig. 2a ) with interpopulation differences ( F ST ) ranging from 0.10 to 0.51. Simulations identified a minimum assay with maximum power using 8 of the highest ranked loci in terms of F ST (between 0.07 and 0.51), which correctly assigned all fish to area of origin, except for one individual identified unambiguously as a North Sea migrant in the Baltic Sea. In a legal framework, it is common practice to evaluate the relative likelihoods of observing the evidence under the prosecution and defence hypothesis (or claims). In this case study, the calculated likelihoods of observing a particular genotype was always more than 6 times higher in the true population of origin than for the second most likely population of origin; for 95% of the cod, it was more than 1,500 times higher, while the median value was 600,000 times higher. 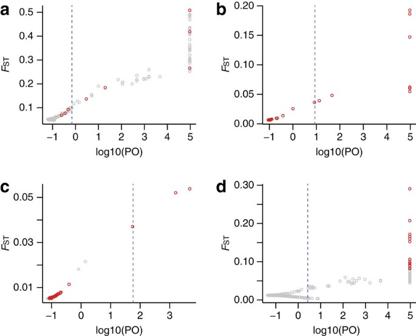Figure 2: Identification of outlier loci. Loci likely to be subject to selection in the four species, using a model-based genome scan approach. Each gene locus (grey circle) is represented by the level of genetic differentiation (FST) and log10 PO of being under selection. Vertical dashed lines mark the threshold corresponding to a false discovery rate of 5%. Loci included in the minimum assays with maximum power are indicated (red circles). (a) Atlantic cod. (b) Atlantic herring. (c) Sole. (d) European hake. Figure 2: Identification of outlier loci. Loci likely to be subject to selection in the four species, using a model-based genome scan approach. Each gene locus (grey circle) is represented by the level of genetic differentiation ( F ST ) and log10 PO of being under selection. Vertical dashed lines mark the threshold corresponding to a false discovery rate of 5%. Loci included in the minimum assays with maximum power are indicated (red circles). ( a ) Atlantic cod. ( b ) Atlantic herring. ( c ) Sole. ( d ) European hake. Full size image Herring One-step genotyping and validation in herring revealed 281 variable SNPs genotyped in 18 Eastern Atlantic samples ( Fig. 1b ). Overall, 16 SNPs were identified as significant outliers. Between Northeast Atlantic and North Sea herring, nine outlier SNPs were identified ( Fig. 2b ). Simulations revealed that the 32 highest ranking SNPs ( F ST between 0.01 and 0.19) could correctly assign 100% of the Northeast Atlantic and 98% of the North Sea herring to their geographic origin (in total 161 out of 163 individuals). The log likelihood ratio between alternative hypotheses of origin, (the prosecutor versus defence claims) revealed that the true population of origin was always more than 3 times more likely (maximum 7 million times more likely) while the median value was 16,800 times more likely. The very few misassigned individuals had low likelihood ratios implicating uninformative genotypes rather than migrant individuals sampled in the other population group. Sole For sole, 27 Atlantic and Mediterranean samples were examined. Within the 16 Atlantic samples ( Fig. 1c ), 19 of 427 SNPs seemed to be influenced by selection. For the Thames/Belgian coast versus Irish Sea/Celtic Sea scenario, three outliers were identified ( F ST values between 0.037 and 0.054). An in silico assay of 50 SNPs showing the highest F ST values (0.005–0.054, Fig. 2c ) correctly assigned 93% (149 out of 160 individuals) to area of origin. The median log likelihood ratio between alternative populations of origin showed that an 'average' individual was more than 60 times more likely in the population of origin even across this very small geographical scale with potentially large population mixing [22] . Hake Hake collections (19 populations) covered Atlantic and Mediterranean basins ( Fig. 1d ). In total, 72 of 395 SNPs were outliers ( Fig. 2d ). 13 high F ST SNPs ( F ST between 0.08 and 0.29) provided 98% (751 of 766 individuals) correct assignment to basin. Fourteen of 15 misassigned individuals originated from western Mediterranean samples (Algerian coast, Malaga) likely to be migrants or the result of admixture with neighbouring Atlantic populations. One individual sampled in the Atlantic was misassigned to the Mediterranean. Excluding likely migrants from the western Mediterranean, 99% of all individuals were assigned unambiguously to basin of origin. Evaluation of the likelihood of alternative hypotheses of origin showed that 95% of all sampled hake were over 500 times more likely to originate from their basin of sampling than to other basins. The policy-led IUU and mislabelling case scenarios demonstrate the large potential for using high differentiation SNPs for assigning individual marine fish to population of origin across a range of geographic scales. For any single assay, the gene-associated SNP framework provides unprecedented levels of assignment power for evaluating hypotheses of fish origin [23] , [24] . For hake, a previous attempt of assigning fish to basin of origin (Atlantic/Mediterranean) using five microsatellites failed due to lack of statistical power [24] . The authors concluded: '...these two geographical stocks cannot be reliably identified from each other neither for fishery forensics nor for commercial traceability'. In addition to the elevated power of assignment, these new SNP-based methods are more readily developed, validated and standardized (because of binary nature), in comparison to other markers such as microsatellites that require extensive inter-laboratory calibration [25] , thereby providing potentially highly valuable legal evidence. Not only, in most cases, can we determine the fit of a genotype to a single population of origin, but, as likelihoods of alternative explanations are bimodal, unequivocal evaluation of the prosecutor versus defence claims is also possible. For the few cases, where unambiguous assignment of individual fish to area of origin was not possible, statistical inferences from a number of individuals can be combined to provide the desired level of certainty. The 'minimum markers with maximum power' are transferable across instruments, requiring limited cross-calibration among laboratories; the approach relies on a centrally accessible SNP database maintained by the European Commission Joint Research Centre. Accordingly, on public release, any potential end-user can create and evaluate in silico assays tailored to specific control and enforcement or product certification scenarios. Typically, forensic authenticity testing examines specific alternative hypotheses of claimed geographical origin rather than the potential origin across the full species' distribution. Thus, targeted assays as presented here are faster, cheaper and more flexible than universal all-purpose SNP arrays. It is now possible to process and genotype several hundred fish per day with assays up to 100 SNPs for less than 25$ per individual in almost any reasonably well equipped molecular genetic laboratory. Finally, design flexibility allows the choice among speed, cost and statistical power, for example, whereas high individual exclusion power is critical in a court of law; genotyping speed can be more essential in real-time spatially based fisheries management. Here rapid genotyping of a few SNP markers in many individuals may provide vital information on the approximate contribution of different populations to a specific marine fishery. With any method, there are potential pitfalls. The gene-associated SNP approach bears the inherent problem of genetic methods that management units are not necessarily equal to biological population units [26] . Thus, different management regulations may be imposed for the same genetic population under different jurisdictions (and vice versa ), leaving genetic methods with reduced discriminatory power. However, these limits to genetic resolution may also reflect ill-defined management areas [26] . Here other methods such as elemental fingerprinting of otoliths or parasite distribution could prove complementary [10] . Likewise, we focussed here on reproductively isolated populations–that is, the fundamental population unit. However, there will be some areas and times of year, where mixed aggregations of individuals from different spawning populations occur and where assigning single individuals to a specific population may provide little information on geographic origin. Here mixed-stock analysis can be applied [27] potentially providing 'mixture signatures' for management areas at certain times. Another special concern is the temporal stability of allele frequencies for genetic markers subject to environmental selection. We expect that most genetic changes will occur over evolutionary timescales; however, if direct or hitch-hiking selection acting on these markers is fast and on-going, allele frequencies in the reference populations could shift. To investigate temporal shifts, analysis of the SNP markers used for the minimum assay developed for cod has been conducted using temporally replicated samples, revealing very small nonsignificant changes in allele frequencies ( P -values between 0.11 and 0.92). 97% of contemporary cod samples correctly assigned to historical samples from the same population and the very few 'misassigned' individuals are likely to represent migrant individuals from other populations ( Fig. 3 ). However, as the functional properties and relationship with environmental changes are unknown for most gene-associated SNPs, validation of the database should be conducted at intervals informed by the biology of the species and local conditions. 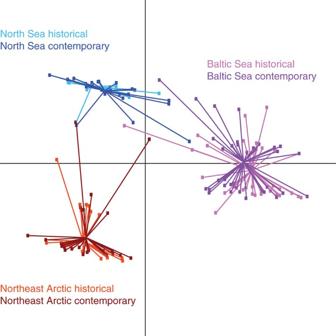Figure 3: PCA plot based on individual genotypes from cod. PCA plot based on individual genotypes from Northeast Arctic, North Sea and Baltic cod, illustrating temporal stability of assignment (6, 4 and 10 years between samples, respectively) for the designated 8 SNP panel. Figure 3: PCA plot based on individual genotypes from cod. PCA plot based on individual genotypes from Northeast Arctic, North Sea and Baltic cod, illustrating temporal stability of assignment (6, 4 and 10 years between samples, respectively) for the designated 8 SNP panel. Full size image The present study examined the application of gene-associated SNPs, which are likely to be affected by adaptive evolution, as high-resolution tools for population traceability to tackle IUU and/or product mislabelling. The issue of SNP-associated gene function in fish has received little attention thus far. However, the many SNPs apparently subject to direct or indirect selection shown here and elsewhere in marine fish [12] , [20] , strongly suggests that populations of marine organisms are genetically adapted to local environmental conditions despite high levels of gene flow. Therefore, the examined SNPs are not mere 'stamp collections [28] ' without biological significance. In many cases, they likely represent functional biological diversity in genes influencing survival and reproduction. Such population diversity, or 'biocomplexity [27] ', underpins functioning, resilience and productivity of marine ecosystems. The 'portfolio effect' of intraspecific biodiversity has been shown to stabilize ecosystem processes and services [29] . It is fortuitous that the adaptive genetic diversity that we aim to conserve underpins the tools that will allow enhanced governance of global fish resources. Sampling Tissue samples (flesh, gills or finclips) of cod ( G . morhua ), herring ( C . harengus ), sole ( S . solea ) and hake (M. merluccius ) were collected on a pan-European scale including additional northwest Atlantic samples for cod ( Supplementary Table S1 ). Sampling was guided by previous genetic and ecological studies indicating population structuring in respective species. Spawning individuals were collected preferably to sample genetic populations. All individuals from an area (population sample) were at all occasions collected on the same cruise. Overall, 85% of the baseline samples collected, including temporal replicates, originated from scientific cruises. The remaining 15% were collected by contracted commercial fishermen on designated cruises. The distribution of samples collected on scientific/commercial cruises was relatively uniform among species with scientific collections constituting 83%, 93%, 87% and 77% for cod, herring, sole and hake, respectively. All samples included in the database were labelled with information on the approach of sampling ( Supplementary Table S1 ). As an additional check of the very unlikely event of any sample mislabelling or substitution (that is, from vessel of sampling to SNP genotype database), patterns of population differentiation among all samples (pairwise F ST ) were evaluated after genotyping. This approach was used to identify any population samples that deviated from the general pattern of population structure established by this or previous studies. However, as expected, no such aberrant population samples were identified. Specific detailed information on individual samples is available at the FishPopTrace database accessible at http://fishpoptrace.jrc.ec.europa.eu/sampling (see also Supplementary Fig. S1) . For cod, samples originated from an extensive tissue bank maintained at the Danish Technical University established from previous studies [30] . SNP discovery and genotyping SNPs for herring, sole and hake were identified through 454 sequencing (Roche 454 GS FLX sequencer) of the transcriptome. Accordingly, as the trancriptome consists of DNA segments transcribed into RNA molecules encoding at least one gene, the SNPs developed here are all gene-associated. Briefly, RNA was extracted from eight individuals from each species collected from four locations across the species range to minimize ascertainment (width) bias due to reduced geographic coverage. SNP discovery was performed by de novo sequence clustering and contig assembly, followed by mapping of reads against consensus contig sequences. 1,536 putative SNPs were selected from each species and included on an Illumina Golden Gate array for a one step validation and genotyping approach. Selection was based on information from the Illumina Assay Design Tool which assigns scores for each SNP based on the probability of them performing well in the genotyping assay, putative intron–exon boundaries within flanking regions of putative SNPs, and a visual evaluation of the quality of contig sequences. From these, 281 (herring), 427 (sole) and 395 (hake) SNPs proved variable with reliable genotyping across population samples. For cod, we used a second generation Illumina 1,536 Golden Gate array with gene-associated loci originating from previous sequencing projects [31] , [32] , [33] . Accordingly, a higher number of these (1,258) could be genotyped reliably across cod samples. Identifying markers likely affected by selection We used a Bayesian likelihood method implemented in BayeScan 2.01 (ref. 34 ) for identifying markers likely to be situated in parts of the genome with one or more genes affected by selection. The method provides posterior odds (PO) as the ratio of the posterior probability of a model of selection versus a neutral genetic model for each locus. In addition, the new version of the program allows for setting 'prior' odds for the two models. In this case, we used the default option that a neutral model was 10 times more likely than a model with selection. Posterior Odds between 32 and 100 (log10(PO)=1.5–2) is considered 'very strong evidence' of selection whereas a PO above 100 is viewed as 'decisive' and finally, a posterior probability of infinity is assigned a log10(PO) of 5. The power of BAYESCAN for detecting markers affected by selection is significantly reduced for comparisons including few samples [34] . Choice of loci For each case, we chose several loci to create our 'minimum assays with maximum power'. Accordingly, the overarching aim was to provide assays with high statistical power, but also sufficiently small to be time and cost effective. The rationale behind this approach is that, in a court of law, the evidence will almost exclusively be weighted in relation to two alternative claimed origins; that is, were the fish caught illegally in area A, as claimed by the prosecutor, or legally in area B, as claimed by the defence? Choice of loci was based on estimates of pairwise genetic differentiation ( F ST ) between samples and subsequent ranking of the loci according to the size of estimate from the outputs of BayeScan. This program employs the multinomial Dirichlet model allowing estimation of population-specific F ST coefficients. To reduce 'high-grading bias' in our assignment tests [35] we first estimated pairwise F ST values and ranked our loci based on half of the individuals from each population as recommended by Anderson [35] . In addition, we did not expect high-grading bias to be particularly prominent when using our concept of application of markers under selection. The very large differences in F ST values, between neutral and loci, identified by the statistical model to be affected by selection found in this study, is unlikely to be caused by sampling error in contrast to rather minute differences in F ST values commonly found among neutral loci. Tightly linked genetic markers represent redundant information, and violate model assumptions used for population assignment that require unlinked loci. Accordingly, we performed linkage analysis among all SNP marker loci, intended for use in the minimum assays. In the case of complete or partial linkage between markers, we excluded the locus with the lowest F ST or lowest genotyping success rate. From the final list of SNP loci included in the four described assays ( Supplementary Table S2 ), we re-genotyped a subset of loci using other genotyping platforms to test for consistency, which was generally high. Assignment procedure Individuals from the baseline case samples were assigned to the population, or in the case of hake to basin (pooled samples within basin), where their multilocus genotype had the highest likelihood of occurring, using the program GeneClass2.0 (ref. 36 ). We employed the Bayesian approach described by Rannala and Mountain [37] to evaluate whether a certain multilocus genotype could occur in (originate from) one or several of the baseline populations using the resampling algorithm described by Paetkau et al . [38] The method, which simulates 10,000 multilocus genotypes per population from baseline allele frequencies, generates expected distributions of likelihoods within populations to compare with estimated individual likelihoods of real genotypes. To evaluate the relative likelihoods of potential alternative origins for a given genotype, we calculated the likelihood ratio of originating from the sampled (home) population divided by the maximum likelihood for any of the other potential alternative populations of origin (L=L_home/L_max_not_home) following Peatkau et al . [38] This approach is equivalent to a standard statistical evaluation of forensic evidence in relation to opposing claims from prosecutor and defence in a court of law; that is, in a potential case of illegal fishing or mislabeling, the likelihoods of observing the genotype in question under the prosecutor and defence hypotheses of origin, respectively, are calculated and evaluated. Values were presented as median and 95% lower percentile values of –log likelihood ratios to illustrate the general high discrimination power of our selected SNP in silico assays. A few of the case scenario individuals had missing single locus genotypes. To maximize sample sizes, they were not excluded for the assignment analyses except for the hake case, where basin samples were plentiful. Incomplete genotypes are expected to reduce the assignment power, so the −log likelihood ratio medians and 95% lower percentiles presented here are expected to be upward biased, that is, more conservative. However, there was no clear indication that misassigned individuals, or individuals assigned with low resolution, were caused by missing genotypic data. Temporal stability To evaluate temporal stability for assignment success with the baseline data, we used temporal genetic data from cod populations. Short-term temporal stability was assessed through tests for genic differentiation using the program GenePop [39] and a principal component analysis (PCA) conducted with the package ADEGENET v.1.2–5 for R [40] of individual genotype data from samples collected from Northeast Arctic cod, North Sea cod and Baltic Sea cod at two time points (4-to-10 years apart). Only the eight loci used in the assignment case for the same populations were used to generate the PCA to visualize the stability of population assignment observed for these specific loci. Accession codes: The sequence data have been deposited in the NCBI dbSNP database under accession codes ss131570937, rs119055455, rs119055265, rs119056441, ss503707782, rs119055013, rs119055651, ss252841231, ss503773365, ss503773368, ss503773371, ss503773374, ss503773376, ss503773379, ss503773381, ss503773384, ss503773385, ss503773388, ss503773391, ss503773394, ss503773396, ss503773398, ss503773401, ss503773404, ss503773406, ss503773408, ss503773411, ss503773414, ss503773416, ss503773418, ss503773421, ss503773423, ss503773426, ss503773428, ss503773431, ss503773434, ss503773436, ss503773439, ss503773441, ss503773444, ss503772144, ss503772147, ss503772150, ss503772153, ss503772155, ss503772157, ss503772160, ss503772163, ss503772166, ss503772168, ss503772171, ss503772174, ss503772176, ss503772179, ss503772181, ss503772184, ss503772187, ss503772190, ss503772192, ss503772195, ss503772197, ss503772200, ss503772203, ss503772206, ss503772209, ss503772211, ss503772213, ss503772216, ss503772218, ss503772221, ss503772224, ss503772226, ss503772228, ss503772231, ss503772234, ss503772237, ss503772240, ss503772243, ss503772245, ss503772247, ss503772250, ss503772253, ss503772255, ss503772258, ss503772260, ss503772263, ss503772266, ss503772269, ss503772271, ss503772273, ss503771126, ss503771130, ss503771134, ss503771137, ss503771139, ss503771143, ss503771146, ss503771148, ss503771150, ss503771155, ss503771157, ss503771160 and ss503771162. How to cite this article: Nielsen, E. E. et al . Gene-associated markers provide tools for tackling illegal fishing and false eco-certification. Nat. Commun. 3:851 doi: 10.1038/ncomms1845 (2012).